Overcurvature describes the buckling and folding of rings from curved origami to foldable tents Daily-life foldable items, such as popup tents, the curved origami sculptures exhibited in the Museum of Modern Art of New York, overstrained bicycle wheels, released bilayered microrings and strained cyclic macromolecules, are made of rings buckled or folded in tridimensional saddle shapes. Surprisingly, despite their popularity and their technological and artistic importance, the design of such rings remains essentially empirical. Here we study experimentally the tridimensional buckling of rings on folded paper rings, lithographically processed foldable microrings, human-size wood sculptures or closed arcs of Slinky springs. The general shape adopted by these rings can be described by a single continuous parameter, the overcurvature. An analytical model based on the minimization of the energy of overcurved rings reproduces quantitatively their shape and buckling behaviour. The model also provides guidelines on how to efficiently fold rings for the design of space-saving objects. Biological phenomena such as the morphogenesis of guts [1] and of some wavy petals and leaves [2] , or technological objects such as stretchable electronic devices [3] , quasi-periodic optical gratings [4] or tridimensionally shaped responsive polymer membranes [5] , [6] , are based on the controlled buckling of thin plates and films. Likewise, rings buckle and fold in saddle shapes: relevant technological, artistic and biological examples have a diameter ranging from a few hundred nanometres to metres, and comprise some of the so-called ‘2-second’ tents and a variety of other popular foldable systems ( Fig. 1a–c ), curved origamis ( Fig. 1d ) [7] , bicycle wheels of excessive spoke tension, released bilayered microrings [8] or confined stiff polymer rings like DNA plasmids in vesicles [9] , [10] . Unlike classical origami that proceeds by discrete steps, the folding of rings results from a continuous evolution of their torsion and curvature. The stored elastic strain energy can then be used for self-deployment from flat, space-saving coils, as in light-weight foldable trekking items. 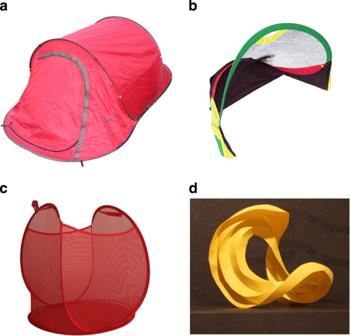Figure 1: Overcurved rings are found in daily life. (a) Foldable ‘2-second’ tent. (b) Foldable football goal. (c) Foldable laundry basket. (d) Author-made curved origami based on a circular crease pattern proposed by Demaineet al.7 Figure 1: Overcurved rings are found in daily life. ( a ) Foldable ‘2-second’ tent. ( b ) Foldable football goal. ( c ) Foldable laundry basket. ( d ) Author-made curved origami based on a circular crease pattern proposed by Demaine et al . [7] Full size image Despite the existence of these tridimensional ring structures at very different length scales and their interest for technological applications and art, they currently lack a direct and generic analytical description capable of simplifying their design. Although the instability of twisted elastic rods and rings is well understood [11] , [12] , the tridimensional shape of closed systems to which a given curvature is pre-set only raised interest recently. Experimental examples are the saddling of bilayered nanorings of various widths [8] and the swelling of elastic polymer sheets with a locally prescribed metrics [5] , [6] , [13] . These experiments were complemented by simulations [14] and theoretical models [15] , [16] , [17] of the buckling of disks or of thin annular surfaces. Analytical results for the buckling of circular rings and arches are available, but only for small and mostly in-plane deformations [18] , [19] , [20] . Analyses of the out-of-plane buckling of rings and arches [18] , [20] , [21] focus on the values of critical loads and do not describe the general shape of strongly buckled systems. Here we concentrate on hoops and rings that fold or adopt saddle shapes when imposed a curvature higher than the one of a circle of identical length. Unlike previous work, we focus on a compact analytical description of the general conformation of these rings using the new notion of overcurvature O , for rings having all cross-sectional dimensions negligible compared with the ring perimeter. Therefore, we first compare experimentally the buckling of closed rings of different cross-sectional shapes, having diameters ranging from 10 micrometres to a few metres. Next, we generate a new family of curves capable of describing the general conformation adopted by buckled rings with a single continuous parameter, the overcurvature O . We then provide a quantitative analytical description of the general shape of overcurved rings of finite cross-section by taking into account the bending and torsional energies. Finally, we use this knowledge to describe how to efficiently fold rings, and demonstrate the folding of a ring into five superposed loops covering a total surface 25 times smaller than the original ring. The model, which is validated on the experimental data, provides an elegant and simple designing tool for overcurved rings as different as a lithographically processed microring or a macroscopic wooden sculpture. A definition of overcurvature The conformation of a buckled or folded closed ring of small cross-section is described by the centre line passing through the centre of gravity of its cross-section, and is represented by a closed curve of equation r ( s ) where s is the arc length coordinate. The centre line can also be defined mathematically by its local curvature κ ( s ) and torsion τ ( s ) [22] . Our analysis will be restricted to untwisted rings having a centre line of constant curvature κ , and a locally variable torsion τ ( s ) that integrates to zero over the ring. Such rings of contour length L are said to be overcurved when the local curvature κ exceeds the curvature of a circle of identical length by a factor O >1, implying the presence of internal stresses. For O =1, the ring is a planar circle of radius R 0 = κ −1 = L /(2 π ). When an additional curvature is applied, An overcurved ring can thus be obtained by increasing its curvature κ while keeping its length L unchanged, or by increasing its length at constant curvature. Experimental illustrations are given in the next section. Experimental overcurved structures We built different overcurved rings of various sizes ( Fig. 2 ), using different materials, cross-sections and overcurvation processes, and classified the different structures according to their pre-set overcurvature O p = Lκ p /(2 π ). The pre-set curvature, κ p , is the curvature that would be spontaneously adopted if the overcurved ring was cut (possibly still involving residual internal stresses as in the second example below). The real curvature κ of the ring is different, due to deformation induced by its closure. Stated otherwise, if a little segment of the ring were to be cut out and allowed to reach mechanical equilibrium, its curvature would be κ p , the pre-set curvature; however, it is forced to sit in a ring of length L >2 π / κ p . Therefore, the segment deforms and takes a local curvature κ taken here as constant. The overcurvature of the ring is O = κL /(2 π ), whereas the pre-set overcurvature is O p = κ p L /(2 π ). 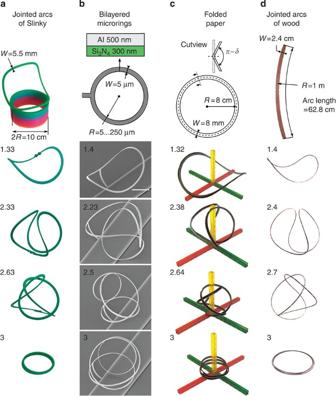Figure 2: Different overcurvation processes can be used to generate overcurved rings. (a) Overcurved closed arcs of a Slinky-like spring (the thicknesstof the beam is 2 mm). (b) Scanning electron microscopy pictures of Al/Si3N4bilayered microrings after release from a silicon oxide substrate (the scale bar is 100 μm). (c) Overcurved rings of paper creased along their curved median line. The coloured rulers are 8 cm in length. (d) Jointed arcs of wood giving rise to human-scale overcurved rings of square cross-section. For these macroscopic systems, gravity starts to affect the shape. The computed or measuredpre-setovercurvaturesOpare indicated in the top left corner of each sub-figure. Figure 2: Different overcurvation processes can be used to generate overcurved rings. ( a ) Overcurved closed arcs of a Slinky-like spring (the thickness t of the beam is 2 mm). ( b ) Scanning electron microscopy pictures of Al/Si 3 N 4 bilayered microrings after release from a silicon oxide substrate (the scale bar is 100 μm). ( c ) Overcurved rings of paper creased along their curved median line. The coloured rulers are 8 cm in length. ( d ) Jointed arcs of wood giving rise to human-scale overcurved rings of square cross-section. For these macroscopic systems, gravity starts to affect the shape. The computed or measured pre-set overcurvatures O p are indicated in the top left corner of each sub-figure. Full size image As first example ( Fig. 2a ), we made buckling rings consisting of connected arcs of Slinky springs. We cut segments of length L in a commercial Slinky spring of central radius R 0 , with L >2 πR 0 . The pre-set curvature κ p is . Then, we connected the two ends of the segments after having tangentially rotated one end to unfold the arc, until the two ends went in contact with the same orientation. This created overcurved rings of pre-set overcurvature O p = L /(2 πR 0 ), which settle in a configuration of minimum energy where forces and moments add up to zero, leading to a balanced state of internal stresses (mechanical equilibrium). This overcurvation process corresponds to varying the length L while keeping the pre-set curvature constant. Typical conformations of the ring are shown in Fig. 2a : as O p increases, the ring progressively bends and folds, then settles into a triple loop for O p =3. A second example is provided by released bilayered microrings ( Fig. 2b ). When two different materials are consecutively deposited to form a linear beam in microfabrication processes, strain mismatch across the layers causes internal stresses that force the beam to bend out-of-plane after release, resulting in a spontaneous curvature κ s (refs 8 , 23 , 24 ). When the same process is used to fabricate a bilayered ring of radius R (before release), the release adds a supplementary curvature κ s perpendicular to the original one (1/ R ), which amounts to overcurve the ring with a pre-set overcurvature ( Supplementary Methods ; Supplementary Fig. S1 ). Bilayered microrings of different radius R were produced by deposition and microlithography [25] , and rectangular beams of identical width and vertical composition were processed in order to determine κ s , which was measured to be 1/90 μ m −1 by scanning electron microscopy. The ring conformations after release are shown in Fig. 2b ; the analogy with the connected arcs of the Slinky spring is obvious, although the close presence of the substrate tends to hinder large deformations during annealing. Creased paper rings are a third example of overcurved structures ( Fig. 2c ). In curved origami, paper is creased along closed curved paths, resulting in the out-of-plane bending of the folding path due to torsion. Simultaneously, the conservation of arc length by the two sides of the crease imposes an increase of the curvature of the crease by a factor O p =1/cos( δ /2) [26] , [27] , where δ is the angle between the normals to the two sides of the crease ( Supplementary Methods ; Supplementary Figs S2 and S3 ; Supplementary equation S19 ). We creased a flat circular ring of paper along its median circle, and adjusted the degree of overcurvature by tuning the crease angle δ and holding it constant. After observations, the paper ring was cut and the number of turns in the formed coil was quantified to compute O p . This overcurvation process corresponds to increasing the local pre-set curvature while keeping the length constant. Finally, to give a human-scale example of overcurved structures, arcs of wood of radius of curvature R =1 m were combined with clamping collars to form closed continuous rings of square cross-section, with different magnitudes of the pre-set overcurvature. Representative images are shown in Fig. 2d and in Supplementary Fig. S4 . The overcurvation scenario is similar for all observed systems: the conformation starts from a circle at O p =1 and buckles to a saddle shape with two pairs of upper and lower lobes for larger pre-set overcurvatures. The opposite lobes of the saddle then overlap close to O p =2.5, and the ring finally debuckles to form a triple-coiled loop for O p =3. All conformations have D 2d symmetry (for creased paper, this holds true only for the crease line). Although some issues are specific to each case, such as the cross-section rotation angle or the formation of wrinkles and lateral creases, the general scenario is identical for these systems, which cover almost five orders of magnitude in spatial scale, and for which the physical origin of overcurving differs sensibly. In the sequel, we concentrate on the general conformation of the centre lines of the rings (or of the crease lines for paper strips), and ignore details such as small wrinkles and lateral creases. Overcurved circles We look for a mathematical description of the centre lines of rings of overcurvature O , by a family of closed curves r ( s , O ) named here overcurved circles. This is done starting from experimental measurements made on creased paper rings and closed arcs of the Slinky spring. For overcurved creased paper rings, we demonstrate in the Supplementary Methods that the curvature of the crease line is constant all over the ring when the width of the paper strip is small enough. This is not generally true for larger strip widths; however, even in this case, the curvature remains constant if the crease angle is held fixed by rigidifying the structure, as was checked experimentally for O p =2.07 ( Supplementary Methods ; Supplementary Figs S5 and S6 ). Likewise, for two overcurved rings made of segments of the Slinky spring, of pre-set overcurvature O p =1.5 and 2.33, the curvature of the centre line was constant within experimental precision (Methods; Supplementary Figs S7 and S8 ). In addition, over each lobe of the overcurved rings, the ends of the curvature vector [22] k ( s )=d 2 r /d s 2 were sitting in the same plane within experimental precision ( Supplementary Fig. S9 ); hence, they belonged to the intersection of a sphere and a plane. Given these observations, we define overcurved circles as tridimensional closed curves having a curvature vector of constant magnitude, with its end lying on the parallel of a sphere for each of the four lobes. Curves of constant curvature with their normal vectors n ( s )= κ −1 k ( s ) lying on a parallel of a sphere are known as Salkowski curves, and can be described parametrically [28] , [29] , [30] . In order to construct overcurved circles, four pieces of Salkowski curves are thus connected while respecting the D 2d symmetry of the problem and ensuring the continuity of the torsion τ ( s ). This can be done by generalizing a procedure recently proposed by Monterde [29] based on previous work by Koch and Engelhardt [31] . The procedure involves constructing a closed and continuous normal indicatrix, or nortrix, which is the locus of the ends of the normal vectors n ( s ), leading to the final curve by double integration with respect to s . Take a right two-sided antiprism of height h with a lateral midsphere of unit radius ( Fig. 3a ). The lateral midsphere of the antiprism is the sphere having the same barycenter as the antiprism, and which is tangent to its lateral edges at midlength. The intersection of the antiprism with its lateral midsphere defines four circles of angular opening φ , where φ is bijectively related to h ( Supplementary equations S34 and S35 ). Two successive intersection circles are tangent, because the lateral edge that separates them is a common tangent. In order to build a nortrix, arcs of these circles are connected by joining either the circular arcs of central angle ω open towards the bases of the isosceles triangles (yellow curve in Fig. 3a ), or the ones of central angle 2 π − ω open to the apexes (blue curve). These two possible paths are continuous to first order because the arcs are tangent. Double integration of any of these two nortrices with respect to arc length generates an overcurved circle containing four lobes; each lobe is a piece of a Salkowski curve having normal vectors n ( s ) making a constant angle φ with respect to the normal to the corresponding side face of the antiprism; the four lobes are related by the rotoinversion axis of the D 2d symmetry group of two antiprisms. The continuity of the nortrix ensures that the final curve is continuous to third order and has a continuous torsion. Hence, the so-defined curves respect all our requirements; their analytical expression is given in the Supplementary Methods ( Supplementary equations S46–S51 ). 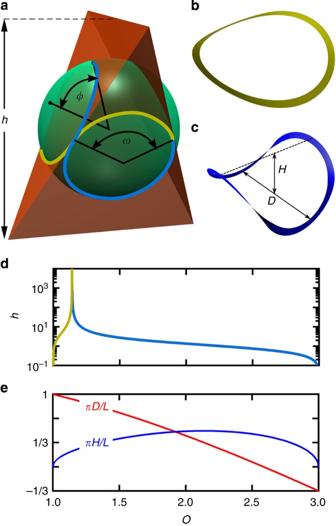Figure 3: Overcurved circles are mathematical curves obtained by double integration of the intersection between a sphere and an antiprism of variable heighth. (a) Intersection between a two-antiprism and its lateral midsphere of unit radius (drawn forφ=0.872 andh=3.108). The two possible paths for the nortrix are indicated in yellow and blue. (b) Conformation of the overcurved circle obtained by double integration of the yellow nortrix of panela(O=1.041). (c) Conformation of the overcurved circle obtained by double integration of the blue nortrix of panela(O=1.443), together with a graphical definition of the distance between the apexes of opposite lobes,D, and the height of the curve,H. (d) Relationship between the height of the two-antiprism and the overcurvature of the resulting overcurved circles. The curves in yellow and blue are related to the two possible paths for the nortrix, displayed with the same colour code in panela. (e) Normalized distance between opposite lobes,πD/L, and height,πH/L, of overcurved circles, versus their overcurvatureO. Figure 3: Overcurved circles are mathematical curves obtained by double integration of the intersection between a sphere and an antiprism of variable height h . ( a ) Intersection between a two-antiprism and its lateral midsphere of unit radius (drawn for φ =0.872 and h =3.108). The two possible paths for the nortrix are indicated in yellow and blue. ( b ) Conformation of the overcurved circle obtained by double integration of the yellow nortrix of panel a ( O =1.041). ( c ) Conformation of the overcurved circle obtained by double integration of the blue nortrix of panel a ( O =1.443), together with a graphical definition of the distance between the apexes of opposite lobes, D , and the height of the curve, H . ( d ) Relationship between the height of the two-antiprism and the overcurvature of the resulting overcurved circles. The curves in yellow and blue are related to the two possible paths for the nortrix, displayed with the same colour code in panel a . ( e ) Normalized distance between opposite lobes, πD / L , and height, πH / L , of overcurved circles, versus their overcurvature O . Full size image The overcurvature O of overcurved circles can be expressed as a function of the height h of the antiprism ( Fig. 3d ); the complete range 1 ⩽ O ⩽ 3 is covered by the blue and yellow paths of Fig. 3a when the height h of the antiprism varies from 0 to ∞ . Conversely, all geometrical parameters ( h , φ and ω ) can be expressed mathematically as functions of O ( Supplementary equations S34, S35 and S53 ). Hence, this geometrical ansatz leads to the generation of a complete family of curves parameterized by O . Figure 3b shows the saddle shapes of overcurved circles for O =1.041 and 1.443, respectively, ( h =3.108). Single-coil and triple-coil flat circles are obtained for O =1 and 3, respectively. Figure 3e presents the normalized height H / L of overcurved circles and the normalized distance between the apexes of their opposite lobes, D / L , versus overcurvature O . Buckled rings Quantitative measurements were performed on rings made of arcs of the commercial Slinky spring, whose conformations proved to be highly reproducible and for which the pre-set overcurvature can be accurately measured. The normalized distance between the apexes of opposite lobes, D / L , averaged over the two pairs of lobes, is plotted versus O p in Fig. 4e (red dots). Two plateaus of constant D / L are observed at the beginning and at the end of the curve, corresponding to flat circular conformations. Between these two plateaus, D / L varies almost linearly with O p . The transition from a flat circle to a saddle defines the buckling overcurvature O b which marks the end of the first plateau, while the transition from the buckled states to a flat triple coil corresponds to the debuckling overcurvature O d , which signals the start of the second plateau. On the plateaus, the rings remain flat and adopt simple circular shapes with well-defined amounts of stored elastic energy dictated by the local curvature κ . Because κ −1 and L evolve proportionally, the overcurvature O remains constant on these plateaus. 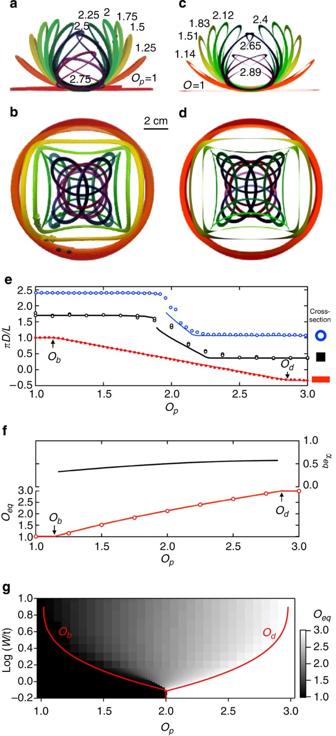Figure 4: Overcurved material rings can be quantitatively described by minimizing their torsion and bending energies. (a,b) Experimental side and top views of overcurved rings made of closed arcs of a commercial Slinky spring for pre-set overcurvaturesOpranging from 1 to 3. (c,d) Corresponding overcurved circles with the overcurvatureOselected in order to reproduce the experimental distanceDbetween the apexes of opposite lobes. The experimental demonstration of the quantitative agreement of the model shape is in the Methods. (e) Comparison between experimental and simulated normalized distancesD/Lbetween the lobe apexes. The circular symbols are the experimental data; the continuous lines are the simulations. The red curve is for closed arcs of a commercial Slinky spring of rectangular cross-section; the black curve (shifted vertically by 0.7) is for closed arcs of a home-made poly(vinyl chloride) spring of square cross-section; the blue curve (shifted vertically by 1.4) is for closed arcs of a polyamide spring of circular tubular cross-section. (f) Computed equilibrium overcurvatureOeq(red curve) and computed equilibrium torsion reduction coefficientαeq(black curve) of closed arcs of the Slinky spring of panele. The open circles are experimental data from panelsaandc. (g) Simulated bidimensional map of the equilibrium overcurvature of closed arcs of a poly(vinyl chloride) ring of rectangular cross-section and of increasing values of widthWversus thicknesst, forpre-setovercurvaturesOp. The red lines are the loci of the bucklingOband debucklingOdovercurvatures. Figure 4: Overcurved material rings can be quantitatively described by minimizing their torsion and bending energies. ( a , b ) Experimental side and top views of overcurved rings made of closed arcs of a commercial Slinky spring for pre-set overcurvatures O p ranging from 1 to 3. ( c , d ) Corresponding overcurved circles with the overcurvature O selected in order to reproduce the experimental distance D between the apexes of opposite lobes. The experimental demonstration of the quantitative agreement of the model shape is in the Methods. ( e ) Comparison between experimental and simulated normalized distances D / L between the lobe apexes. The circular symbols are the experimental data; the continuous lines are the simulations. The red curve is for closed arcs of a commercial Slinky spring of rectangular cross-section; the black curve (shifted vertically by 0.7) is for closed arcs of a home-made poly(vinyl chloride) spring of square cross-section; the blue curve (shifted vertically by 1.4) is for closed arcs of a polyamide spring of circular tubular cross-section. ( f ) Computed equilibrium overcurvature O eq (red curve) and computed equilibrium torsion reduction coefficient α eq (black curve) of closed arcs of the Slinky spring of panel e . The open circles are experimental data from panels a and c . ( g ) Simulated bidimensional map of the equilibrium overcurvature of closed arcs of a poly(vinyl chloride) ring of rectangular cross-section and of increasing values of width W versus thickness t , for pre-set overcurvatures O p . The red lines are the loci of the buckling O b and debuckling O d overcurvatures. Full size image Figure 4a show the conformations of Slinky spring rings with pre-set overcurvature O p between 1 and 3. The conformations of overcurved circles of overcurvature O selected to have the same values of D / L are reproduced in Fig. 4c . All the experimentally observed conformations can be qualitatively covered by the geometrical ansatz. The ( x , y , z ) coordinates of the centre line of overcurved Slinky rings of pre-set overcurvature O p =1.5 and 2.33 were also measured (Methods; Supplementary Fig. S7 ). An excellent agreement was found with the coordinates of overcurved circles of overcurvature O =1.54 and 2.5, respectively, confirming the quantitative ability of the theoretical model to represent the tridimensional shape of overcurved rings. A reasonably good agreement was also found for measurements performed on creased paper rings ( Supplementary Fig. S6 ). However, O ≠ O p ; therefore, a relationship between these two parameters still needs to be derived to quantitatively analyse the shape of overcurved rings. In addition, the origin for the buckling and debuckling plateaus has to be explained. This requires taking into account the variations of the bending and torsional energies of the ring, depending on its cross-sectional shape and stiffness. Consider a ring of pre-set curvature κ p in the undeformed, flat state. When a portion of length is connected to create an overcurved ring, internal stresses build up. Therefore, the local curvature changes to κ ≠ κ p , and the ring buckles out-of-plane to decrease the bending energy. Simultaneously, a torsional deformation τ m ( s ) appears, where τ m ( s ) is the gradient of rotation of the cross-section along the centre line [32] . Given the good agreement between experimental conformations and the shape of overcurved circles, we postulate that the final conformation of the buckled ring can be described by an overcurved circle of overcurvature O = Lκ /(2 π )≠ Lκ p /(2 π )= O p , and that the mechanical torsion of the ring is proportional to the mathematical torsion of the centre line: τ m ( s )= ατ ( s ) with α ⩽ 1. Then, the torsional and bending energies of the ring can be expressed as mathematical functions of the pre-set overcurvature O p , actual overcurvature O and torsion relaxation coefficient α , in addition to geometrical and material parameters ( Supplementary Discussion and Supplementary equations S2, S4 and S5 ). Numerical minimization with respect to both O and α of the total energy of the ring provides the equilibrium overcurvature O eq and the equilibrium torsion reduction coefficient α eq , corresponding to a given pre-set curvature O p . These equilibrium parameters were computed for the poly(vinyl chloride) ring made of arcs of the commercial Slinky spring of rectangular cross-section (geometrical parameters are in the Supplementary Table S1 ). The predicted dependence of O eq on O p is compared in Fig. 4f to the experimental data (taken from Fig. 4a ), showing excellent agreement. From the knowledge of O eq , the distance D between the apexes of opposite lobes can be computed using the relationships for overcurved circles. The comparison of experimental and predicted D ( Fig. 4e , red line) indicates a perfect quantitative agreement between theory and experiment. When D tends to zero, there should be a slight perturbation of the shape due to the excluded volume of the ring. This perturbation is too small to be noticed for small cross-sectional dimensions compared with the radius of curvature of the undeformed ring. The predicted effect of a relative change of cross-section dimensions on the equilibrium overcurvature is shown in Fig. 4g , for the case of a rectangular cross-section of width W and thickness t . The equilibrium overcurvature O eq does not depend strongly on the nature of the material of the ring, because the only material constant of relevance in the energy minimization is 1/(1+ν), which typically varies from 0.67 to 0.83 for most materials ( ν is the Poisson ratio). Three regimes can be observed, depending on the anisotropy W / t of the cross-section. For horizontally elongated cross-sections ( W / t ⩽ ∼ 1.05), the stable state is the flat ring ( O eq =1) when the pre-set overcurvature is below the buckling overcurvature O b ; above the debuckling overcurvature O d , the stable state is the triple-coil ring ( O eq =3); in-between these extreme values, the conformation varies continuously as a function of the pre-set overcurvature, sampling all possible values between 1 and 3. In contrast, for vertically elongated cross-sections ( W / t ⩽ ∼ 0.78), the stable state is the flat ring for pre-set overcurvatures <2; for larger pre-set overcurvatures, the stable state is the triple-coil ring. There is thus no continuous conformational change allowing us to pass from one state to the other. Accordingly, when increasing lengths of arcs of a home-made poly(vinyl chloride) spring having W / t =0.5 were connected in a ring by counter rotation of the arc, the system never transited to the triple-coil state. Instead, it remained in the flat single-coil ring metastable state, then buckled in-plane (wrinkling) until crazing and failure happened. For intermediate values of the cross-section anisotropy, the transition between the two plateaus has a mixed character, and metastable states exist: the full analysis is provided in the Supplementary Discussion and Supplementary Figs S10 and S11 . Experiments were performed in this regime on a home-made poly(vinyl chloride) of square cross-section ( Fig. 4e , black) and on a commercial polyamide spring of circular tubular cross-section ( Fig. 4e , blue). The model again reproduces very well the lengthening of the pre- and de-buckling plateaus, as well as the location of the transition and its asymmetry. The small deviations between model and experiment are due in part to the fact that we connected arcs of helices (springs), and not true arcs of circles; therefore, a pre-torsion exists in the flat states that contributes to a slight decrease of the length of the debuckling plateau. Furthermore, for the triple-folded side, excluded volume effects also contribute to disfavour the flat state. Limited plastic deformation of the arcs after straining also explains the deviations between experiment and model. How to fold a ring Although the previous section concentrated on systems of constant pre-set curvature κ p and increasing length L , the folding of rings corresponds to increasing the pre-set curvature while keeping the length of the ring constant. This is the operation performed when, for example, folding the ‘2-second’ tent of Fig. 1a . Because equilibrated ring conformations correspond to overcurved circles, the folding path of least resistance involves forcing the ring to follow the different conformations of overcurved circles of increasing O ; therefore, the notion of overcurvature proves useful for the folding of rings as well. Folding a ring in three loops thus consists of making four lobes that are folded as shown in Fig. 5a . Folding rings will be easier when the cross-sectional shape is selected so as to favour the existence of a continuous set of equilibrated conformations between the initial ring shape and the triple coil: rings of rectangular cross-section are thus easier to fold when they have a larger cross-sectional anisotropy W / t ( Fig. 4g ). Note that the spontaneous unfolding of a folded ring does not follow the folding path of least resistance; instead, it follows the path of steepest energy gradient, that might be quite different and would be worth exploring further. 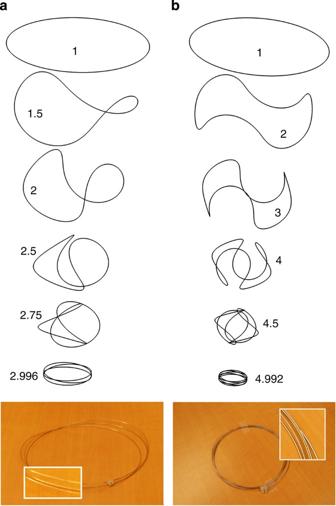Figure 5: How to fold a ring in an odd number of loops. (a) Successive conformations of the ring for three final loops, corresponding to the path of least resistance. The numbers are the overcurvatures. The bottom picture is an experimental realization, where the starting ring was made by bending a steel wire of circular cross-section (1 mm diameter) in a hoop of 1 m diameter. (b) Successive conformations of the ring for five final loops. Figure 5: How to fold a ring in an odd number of loops. ( a ) Successive conformations of the ring for three final loops, corresponding to the path of least resistance. The numbers are the overcurvatures. The bottom picture is an experimental realization, where the starting ring was made by bending a steel wire of circular cross-section (1 mm diameter) in a hoop of 1 m diameter. ( b ) Successive conformations of the ring for five final loops. Full size image An interesting generalization of the theory presented above can be used to find how to fold a ring into a larger number of untwisted loops. It involves taking as nortrix the intersection of a unit midsphere with the side faces of a right m -antiprism, instead of a two-antiprism ( Supplementary Fig. S12 ). The resulting overcurved circle has D m d symmetry and is made of 2 m lobes (arcs of Salkowski curves); it folds into (2 m –1) loops. The complete description is in the Supplementary Methods and Supplementary Table S2 . An example of path to follow to fold a ring into five loops is shown in Fig. 5b ( m =3), together with the experimental example of a ring folded along such a pathway. This peculiar folding corresponds to reducing the diameter by a factor of 5, and therefore the total surface of the ring by a factor of 25, which is a substantial gain in compactness. Whether folding a ring in an even higher number of loops is possible depends on the mechanical characteristics of the ring, the dimensions of its cross-section and its initial pre-set curvature. The excluded volume is likely to make folding more difficult for higher values of m . The analysis presented here is not complete and relies on two assumptions. The first one is the constancy of curvature over the rings, which we demonstrated for creased paper rings of small strip width. For the other studied systems, it remains an hypothesis, which we validated by experimental observations. Further work should concentrate on delineating its conditions of validity; it is likely to break down for systems of larger cross-section. The second assumption is that each lobe of an overcurved ring is a segment of a Salkowski curve. This hypothesis was also validated by experimental measurements, and proved to be mathematically convenient because it allowed us to provide an analytical approximate solution to a non-trivial buckling problem. However, its experimentally demonstrated validity still lacks a compelling reason. Despite these shortcomings, our solution is already able to represent accurately the general shape of the rings and to connect together a series of systems, as well as relating ring buckling and ring folding. Interestingly, the mathematical curves used to model overcurved rings form a complete set of curves parameterized by m and O , which might prove useful for solving other problems of physics of D m d symmetry. Furthermore, the geometrical construction used to generate overcurved circles could be generalized to other more complex systems, including foldable systems containing hinges allowing the total twist to be non-zero. Although our approximate solution does not result from solving instability equations, it provides a simple, quantitatively accurate and analytical method for choosing a pre-set overcurvature O p and the cross-sectional dimensions, leading to a desired overcurved conformation. Therefore, it should find widespread usage for a series of scientific problems, such as the folding of plasmid DNA, the self-folding of rings in tridimensional micro-devices or the compaction of deployable items. In addition, it provides rules for designers and origamists for reaching novel complex shapes; finally, and maybe most importantly, it explains to hikers how to fold some popup tents as fast as they can be deployed. Construction of overcurved rings made of arcs of a Slinky spring Segments of various length were cut in a commercial ‘rainbow’ Slinky spring of 100 mm diameter, with a cross-section of 5.5 mm width and 2 mm thickness. After tangential rotation and alignement, the two ends of the segments were connected by two small M2 bolts separated by 1 cm along the central line of the segments. This prevented the two ends from twisting with respect to each other. Fabrication of overcurved microrings Bilayered microrings were produced by microlithography as reported before [25] , with a top 500-nm thick aluminium layer resting over a 300-nm thick layer of silicon nitride. The cross-sectional width of the rings was 5 μm, and their diameter 2 R ranged from 10 to 500 μm by 2.5 μm steps. Rectangular beams of identical width and vertical composition were also made in order to determine the spontaneous curvature after release. Fabrication of overcurved paper rings of constant crease angle In order to fix the crease angle for paper rings, we progressively impregnated the crease with cyanoacrylate glue, while moving and pinching the crease with tweezers to keep the distance between the edges of the crease constant. This was done for the samples displayed in Fig. 2 . Another method is to use small paper standoffs that are folded and glued in order to fix the distance between the edges of the crease, as described in the Supplementary Methods and Supplementary Fig. S5 . Construction of macroscopic overcurved rings made of arcs of wood Wooden sculptures were made by joining 2 n arcs of wood of rectangular cross-section (width W =24 mm, thickness t =12 mm), having a radius of curvature R 0 =1 m and an arc length L a =62.8 cm (36° of angular opening). The arcs were stacked in two layers, with the arcs in the top layer being translated azimuthally by L a /2 compared with the underlaying layer, like bricks in a wall. The structure was held by clamping collars to form closed continuous rings of square cross-section (width W , thickness 2 t ). The pre-set overcurvature O p = nL a /(2 πR 0 ). Supplementary Fig. S4 is a picture of one of the macroscopic wooden sculptures realized; the arcs of the sculpture were first assembled while not tightening the clamping collars to allow for some flexibility. After the ring was assembled, the bolts were tightened, which resulted in the spontaneous formation of its tridimensional shape. Mathematical construction of an overcurved circle of overcurvature O Given a value of O , the corresponding ω and φ are computed numerically by the Supplementary equations S35 and S53 , and one lobe of the final curve is generated using the t -parameterized equations of Salkowski curves ( Supplementary equations S46–S48 ) by varying t between − ω /2 and ω /2. The other lobes are obtained by Supplementary equations S49–S51 . Spatial rescaling by multiplication of all coordinates by a factor λ can then be applied if needed, with the curvature κ and torsion τ ( s ) of the curve being thereby multiplied by 1/ λ . Validation on Slinky springs of the hypotheses used to build the mathematical model The shape of the centre line of overcurved rings made of closed segments of a Slinky spring was determined by measuring with a ruler (precision 0.5 mm) the ( x , y , z ) coordinates of two rings of 1.5 and 2.33 pre-set overcurvature O p , respectively. This Slinky ring was of 48 mm central radius, and had a rectangular cross-section (2 × 5.5 mm 2 ) with the longer side aligned along the radius of the ring (before overcurvation). Supplementary Fig. S7 presents the recorded experimental values (circles), together with the theoretical prediction for overcurved circles of 1.54 and 2.5 overcurvature O , respectively. The agreement is extremely good, testifying for the capability of the model to represent quantitatively the centre line of overcurved rings and therefore their general conformation. The difference between the pre-set overcurvature O p and the real overcurvature O is due to the deformation of the ring resulting from its closure. The curvature vector of the experimental centre line was computed by double differentiation with respect to arc length, after a slight spline smoothing was applied. Supplementary Fig. S8 shows the computed components of the curvature vector as well as its magnitude κ . When O p =1.5, κ =0.0208, mm with a s.d. of 0.002 mm (measured for 55 equidistant points along the arc); when O p =2.33, κ =0.0218, mm with a s.d. of 0.001 mm (measured for 57 equidistant points along the arc). The experimental error bar on the curvature was also estimated by considering that the distances were measured with an optimistic precision of 0.25 mm, and that errors during differentiation add up in a root-mean-square fashion as is the case for gaussian probability distributions; this provides estimated errors on the curvature of ±0.0036, mm −1 and ±0.0016, mm −1 for O p =1.5 and 2.33, respectively. In both cases, because the estimated error is larger than the s.d. of the measurements, the curvature can be considered to be constant within experimental precision, indicating that the extremities of the curvature vectors of an overcurved ring can be taken to lie over a sphere. Although the limited precision of the doubly differentiated experimental data prohibits to exclude the possible existence of small oscillations of the curvature about its average value [16] , these oscillations—if any—have no perceptible practical consequence for the general conformation of the centre line of the rings as shown in the Supplementary Fig. S7 , where the simulation is obtained assuming the curvature to be constant. Finally, the trajectory of the extremity of the curvature vector, projected over the vertical bisecting plane of a lobe, was computed ( Supplementary Fig. S9 ). The data from four lobes were superimposed for each graph, in order to increase the information content. For the two rings tested, all points aligned within experimental precision, demonstrating that the curvature vector associated to each lobe maybe considered as belonging to a plane. Because the end of the curvature vector also belongs to a sphere, it follows—within experimental precision—that the end of the curvature vector of one lobe describes an arc of a circle and belongs to the intersection of a sphere with a plane. Therefore, the curvature vector also makes a constant angle with respect to the line passing by the centre of the circle and perpendicular to the plane to which the end of the curvature vector belongs. This demonstrates experimentally the validity of the hypotheses used to construct the nortrix of overcurved rings, whose construction is fully described in the Supplementary Methods . How to cite this article: Mouthuy, P-O. et al . Overcurvature describes the buckling and folding of rings from curved origami to foldable tents. Nat. Commun . 3:1290 doi: 10.1038/ncomms2311 (2012).